Methane production by phosphate-starved SAR11 chemoheterotrophic marine bacteria The oxygenated surface waters of the world’s oceans are supersaturated with methane relative to the atmosphere, a phenomenon termed the ‘marine methane paradox’. The production of methylphosphonic acid (MPn) by marine archaea related to Nitrosopumilus maritimus and subsequent decomposition of MPn by phosphate-starved bacterioplankton may partially explain the excess methane in surface waters. Here we show that Pelagibacterales sp. strain HTCC7211, an isolate of the SAR11 clade of marine α-proteobacteria, produces methane from MPn, stoichiometric to phosphorus consumption, when starved for phosphate. Gene transcripts encoding phosphonate transport and hydrolysis proteins are upregulated under phosphate limitation, suggesting a genetic basis for the methanogenic phenotype. Strain HTCC7211 can also use 2-aminoethylphosphonate and assorted phosphate esters for phosphorus nutrition. Despite strain-specific differences in phosphorus utilization, these findings identify Pelagibacterales bacteria as a source of biogenic methane and further implicate phosphate starvation of chemoheterotrophic bacteria in the long-observed methane supersaturation in oxygenated waters. The simplest of all hydrocarbons, methane (CH 4 ), is a potent greenhouse gas that has >20-fold more warming potential than carbon dioxide, making an understanding of its sources and sinks important for global climate models (reviewed in Valentine [1] ). Canonical microbial methanogenesis pathways operate under strictly anaerobic conditions [2] , such that methanogenesis is not favoured in marine surface waters where oxygen is abundant. Historically, the only known sites of classical methanogenesis in the surface ocean were the anaerobic microenvironments of faecal matter and the guts of certain fish or plankton [3] , [4] . Yet, CH 4 profiles in the open ocean show subsurface maxima associated with the pycnocline (density, σ t =25.2–25.9; 50–200 m) where CH 4 is generally supersaturated in relationship to atmospheric equilibrium [5] , [6] . How this methane comes to be produced in oxygenic water masses is the basis of a phenomenon coined the ‘oceanic methane paradox’ [7] , which is particularly intriguing given that the isotopic composition of subsurface CH 4 maxima is inconsistent with that of anaerobic microenvironments [8] . An alternate hypothesis has been proposed: CH 4 is produced when marine microorganisms use methylphosphonic acid (MPn) as a resource for phosphorus (P) [9] . Several lines of evidence support this ‘aerobic methane production’ hypothesis: (i) the C–P lyase enzyme complex catabolizes MPn to CH 4 , releasing phosphate (P i ) that can be used for growth [10] , [11] (reviewed in White and Metcalf [12] ); (ii) C–P lyase gene sequences are present (sometimes abundant) in marine environments [13] , [14] , [15] , [16] , [17] ; (iii) natural seawater samples incubated with MPn release CH 4 [9] , [17] ; (iv) biosynthesis of MPn by Nitrosopumilus maritimus SCM1, a member of the ubiquitous and abundant Marine Group I (MGI) archaea was recently demonstrated [18] ; and (v) ca. 0.6% of microbes in marine surface communities contain genes encoding the MPn synthase [18] . Taken together, these findings suggest the observed CH 4 supersaturation can be explained by the natural synthesis of MPn and subsequent hydrolysis for purposes of P nutrition by marine plankton. For this process to act as a substantial source of CH 4 , there must be an ecophysiological niche for MPn utilization in the oxygenic surface ocean. Isolated cultures of Escherichia coli , Pseudomonas spp. and other heterotrophic bacteria [10] , [12] , as well as marine autotrophs such as Trichodesmium [19] , have been shown to use MPn as a sole P source. In these organisms, MPn degradation proceeds via the C–P lyase pathway and is induced by P i starvation [12] , [20] , [21] , [22] , [23] . Building on these findings, studies by Karl et al. [9] and Martínez et al. [17] showed that when surface seawater is amended with glucose and a nitrogen source (to stimulate P i -limiting conditions), MPn hydrolysis and CH 4 production proceeds at rates that scale inversely with the addition of exogenous P i . The authors implicate a combination of heterotrophic marine bacteria, together with natural assemblages of Trichodesmium spp., as drivers of this metabolism [9] , [17] . These findings are consistent with studies of gene expression [23] and methane production [24] in Trichodesmium erythraeum IMS101 that show induction of C–P lyase genes under P starvation and subsequent methane production from MPn. Although these experiments provide definitive evidence for potential MPn utilization in the surface ocean, they do not necessarily address the CH 4 supersaturation observed at the pycnocline, nor the organism(s) responsible for production of excess CH 4 in these deep layers of the euphotic zone. It seems unlikely that the activity of large buoyant genera such as Trichodesmium can wholly explain the subsurface CH 4 features given that Trichodesmium are largely observed within or at the base of surface mixed layer [25] , [26] and that CH 4 supersaturation has also been observed outside of the subtropical gyres [27] . Alternately, observations of CH 4 maxima below the surface mixed layer and the lack of diurnal variation of these CH 4 levels [6] point to heterotrophic organisms as probable contributors to CH 4 production—provided a steady source of MPn is available and that environmental conditions favour the utilization of dissolved organic phosphorus (DOP). Consistent with the hypothesis that P-starved heterotrophic bacteria produce CH 4 , members of marine Vibrionales and Rhodobacterales expressed C–P lyase genes in P-limited mesocosm studies that, when amended with MPn, also generated CH 4 (ref. 17 ). The SAR11 clade of oligotrophic α-proteobacteria ( Pelagibacterales ) are the numerically dominant chemoheterotrophic cells in marine euphotic zones worldwide [28] . Environmental and laboratory studies have elucidated the forms of dissolved organic matter Pelagibacterales bacteria use, including reduced sulphur compounds, amino acids, one-carbon compounds, organic acids (reviewed in Tripp [29] ) and vitamin precursors [30] . Despite a high degree of genomic conservation between Pelagibacterales genomes [31] , strategies for acquiring P appear to vary between Pelagibacterales isolates. For example, compared with the northeast Pacific Ocean isolate, ‘ Candidatus Pelagibacter ubique’ strain HTCC1062 (str. HTCC1062, herein), the genome of Pelagibacterales sp. strain HTCC7211 (str. HTCC7211), isolated from the North Atlantic Ocean in the Sargasso Sea [32] , encodes for additional proteins involved in organophosphorus transport (PhnCDEE 2 ) [20] and phosphonate utilization (PhnGHIJKLNM), suggesting that the two organisms have evolved different adaptive strategies for P acquisition related to niche partitioning [14] . Here, building on these genomic insights we test the hypothesis that Pelagibacterales chemoheterotrophic bacteria encoding the C–P lyase complex produce CH 4 from MPn when P i starved. We show that str. HTCC7211 produces CH 4 from MPn in proportions stoichiometric to P demand. Moreover, we present rates of CH 4 production under ideal growth conditions, together with the genetic response to P starvation in the Pelagibacterales . These data suggest Pelagibacterales are one of the leading contributors to CH 4 dynamics in P i -deficient oligotrophic gyres. The capacity of Pelagibacterales strains HTCC1062 and HTCC7211 to grow on multiple alternate P sources, including phosphite, phosphonates and phosphate esters, was tested. Strain HTCC1062 grew on P i and did not use added DOP ( Fig. 1 ). In contrast, str. HTCC7211 used a broad range of alternate compounds for P nutrition, including P esters (phosphoserine, glucose 6-phosphate and ribose 5-phosphate), phosphonates (2-aminoethylphosphonic acid and MPn) and reduced inorganic P (phosphite) ( Fig. 1 ). In all cases, diauxic growth was observed when str. HTCC7211 cells were grown with an alternate P source ( Fig. 2 ); this growth pattern is presumably related to a transition from growth on P i to growth on organic P resources as has been described for other organisms [33] , [34] . There was no significant difference in negative control (no P i added) cell yields and the cell yields attained when glucose 6-phosphate, ribose 5-phosphate, MPn, 2-AEP and phosphoserine were supplied to str. HTCC1062 ( Fig. 1 ). We presume that this is an indication that abiotic P i release from these compounds is negligible. The increased str. HTCC1062 cell yields when grown with phosphite as a sole source of P could result from (i) trace amounts of phosphate; (ii) abiotic conversion (oxidation) of phosphite to phosphate; or (iii) the ability of str. HTCC1062 to enzymatically oxidize phosphite to phosphate via an unknown mechanism. At this time we do not have evidence that supports one of these possibilities over the other. 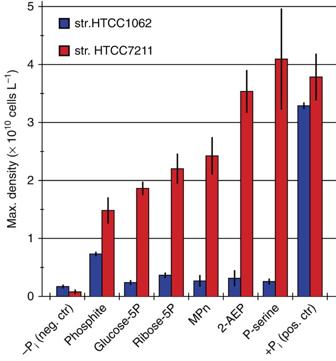Figure 1: P-source utilization byPelagibacteralesstrains HTCC1062 (blue) and HTCC7211 (red). Bar height is the mean of the maximum density achieved for biological replicates±1.0 s.d. (n=3). Piwas supplied as NaH2PO4in the positive control. Growth medium was not amended with Piin the negative control. Remaining treatments had 1.0 μM of P source added. Figure 1: P-source utilization by Pelagibacterales strains HTCC1062 (blue) and HTCC7211 (red). Bar height is the mean of the maximum density achieved for biological replicates±1.0 s.d. ( n =3). P i was supplied as NaH 2 PO 4 in the positive control. Growth medium was not amended with P i in the negative control. Remaining treatments had 1.0 μM of P source added. 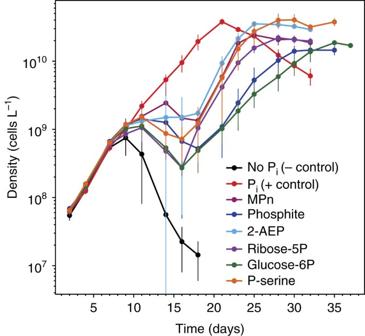Figure 2: Diauxic growth ofPelagibacterales sp. str. HTCC7211 on alternate phosphorus sources. Points are the mean densities of biological replicates±1.0 s.d. (n=3). Each alternate phosphorus compound was supplied at a final concentration of 1.0 μM. Piwas supplied as NaH2PO4in the positive control. Growth medium was not amended with Piin the negative control. Remaining treatments had 1.0 μM of P source added. Cell inoculum was previously grown on Pi. Full size image Figure 2: Diauxic growth of Pelagibacterales sp . str. HTCC7211 on alternate phosphorus sources. Points are the mean densities of biological replicates±1.0 s.d. ( n =3). Each alternate phosphorus compound was supplied at a final concentration of 1.0 μM. P i was supplied as NaH 2 PO 4 in the positive control. Growth medium was not amended with P i in the negative control. Remaining treatments had 1.0 μM of P source added. Cell inoculum was previously grown on P i . Full size image The genetic basis for the P source utilization patterns observed for each strain was investigated at a transcriptional level using DNA microarrays. Time-course experiments showed that P i -starved str. HTCC1062 cultures rapidly induced expression of pstSCAB , encoding the high-affinity transport system ( Fig. 3 ). Individual pst genes were upregulated 2.4- to 3.6-fold 4 h after the onset of P i starvation and 9.1- to 27.9-fold 38 h after the onset of P i starvation ( Fig. 3 and Supplementary Tables 1–3 ). A concomitant upregulation of global stress-response genes (including recA , lexA and umuD ) and downregulation of ribosomal protein transcripts (including rpsB , rpsP , rpsK , rpsS , rplB and rplC ) suggested that P i depletion is treated as a global stressor in str. HTCC1062 ( Supplementary Tables 2–3 ). P i starvation of str. HTCC7211 induced expression of genes encoding the organophosphorus ABC transporter ( phnCDEE 2 ; 7.3- to 21.8-fold) and the C–P lyase ( phnGHIJKLM ; 2.1- to 7.3-fold) ( Fig. 3 and Supplementary Tables 4 and 5 ). Genes encoding str. HTCC7211’s high-affinity P i transporter pstSCAB were also upregulated, but to a lesser degree (3.2- to 3.7-fold) than the organophosphorus transporter. In contrast to str. HTCC1062, stress-response genes were not differentially regulated in str. HTCC7211. 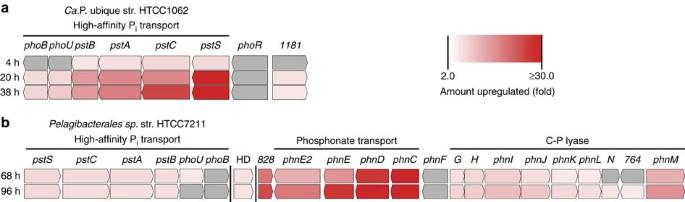Figure 3: Comparative genomics of select P acquisition-related gene expression in Pi-starved cell suspensions ofPelagibacteralesstrains HTCC1062 (a) and HTCC7211 (b). The time elapsed since the onset of resuspension is shown to the left of each gene row. Vertical lines between genes inbrepresent a lack of genomic synteny. Genes shaded grey were not significantly differentially expressed. Gene names, annotations and actual expression values are listed inSupplementary Tables 1–5. 1181, SAR11_1181; HD, H-D Hydrolase; 828, PB7211_828; G,phnG; H,phnH; N,phnN, 764, PB7211_764. Figure 3: Comparative genomics of select P acquisition-related gene expression in P i -starved cell suspensions of Pelagibacterales strains HTCC1062 (a) and HTCC7211 (b). The time elapsed since the onset of resuspension is shown to the left of each gene row. Vertical lines between genes in b represent a lack of genomic synteny. Genes shaded grey were not significantly differentially expressed. Gene names, annotations and actual expression values are listed in Supplementary Tables 1–5 . 1181, SAR11_1181; HD, H-D Hydrolase; 828, PB7211_828; G, phnG ; H, phnH ; N, phnN , 764, PB7211_764. Full size image Although str. HTCC7211 used the P-esters glucose 6-phosphate, ribose 5-phosphate and phosphoserine for growth, the mechanism of utilization is unclear and might involve a novel phosphatase. Genes encoding recognized bacterial alkaline phosphatases, commonly associated with P-ester hydrolysis ( phoA , phoD and phoX ) [35] , are absent from the str. HTCC7211 genome. We speculate that str. HTCC7211 encodes a novel phosphatase, with a broad substrate range, that may explain the observed utilization of P esters. The HD-hydrolase (‘HD’ in Fig. 3b ), induced by P i depletion, is a member of a large family of metal-dependent phosphohydrolases [36] and may act on P esters to release P i . Interestingly, a second gene ( PB7211_828 ; ‘828’ in Fig. 3b ), divergently transcribed downstream of phnE 2 and annotated as a ‘hypothetical protein’, was upregulated 12- to 15-fold in P i -deplete conditions. Although PB7211_828 is unique to str. HTCC7211 (a so-called ORFan [37] ), peptides mapping to PB7211_828 were identified in Sargasso Sea metaproteomes [38] , suggesting an important role in the response to P stress. Given its genomic context adjacent to an organophosphate transporter ( phnCDEE 2 ) and strong upregulation under P i -deplete conditions, we postulate that PB7211_828 may be involved in P-ester hydrolysis. CH 4 is a product of MPn hydrolysis by P i -starved str. HTCC7211 cells. When synthetic growth medium [39] (without added P i ) was amended with excess MPn (10 μM), str. HTCC7211 produced CH 4 ( Fig. 4a ) concomitantly with cell growth ( Fig. 4b ). CH 4 was not produced when cells were grown with P i additions ( Fig. 4a ) and CH 4 production from MPn was repressed when cells were grown in the presence of MPn and P i ( Table 1 ). Mass balance confirmed this observation: 1.29±0.18 μM CH 4 (mean±s.d. ; n =3; presumably from the catabolism of 1.29±0.18 μM MPn) was produced over the course of the 36-day incubation, plus 8.47±0.21 μM residual DOP (mean±s.d. ; n =3) measured at the end of the experiment, account for the full complement of added MPn (10 μM). In culture, cell-normalized CH 4 production was 15.2±0.04 amol CH 4 per cell (mean±s.d. ; n =3) at an average rate of 0.42 amol CH 4 per cell per day. For comparison, the P quota of MPn-grown str. HTCC7211 was 10.04±0.02 amol per cell ( Table 2 ), suggesting that the hydrolysis of MPn exceeded the cellular P demand under these ideal growth conditions. At high P source concentrations (>67 nM), significant growth rate differences were observed between the MPn and P i treatments (0.29±0.00 and 0.36±0.01 per day, respectively; t -test P -value: 0.000007, n =6) ( Table 3 ). Overall growth rates were slower at lower concentrations (<67 nM) of MPn or P i but did not differ significantly as a function of P source (0.22±0.02 and 0.24±0.04 per day, respectively; t -test P -value: 0.35, n =6) ( Table 3 ). 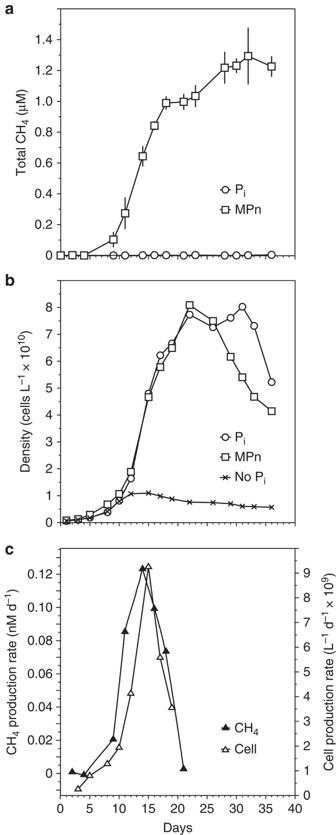Figure 4:Pelagibacteralesstr. HTCC7211 produces methane when Pistarved. (a) Total CH4concentration in sealed bottles fromPelagibacterales sp.str. HTCC7211 cultures grown with MPn or Pi. Points are the mean CH4concentration±1.0 s.d. (n=3) (b) Cell densities from bottles ofPelagibacterales sp.str. HTCC7211 cultures grown with no Pi, MPn or Pi. Cell counts for each treatment were obtained from single bottles used solely for cell counts. (c) The CH4production rate (change in CH4concentration per day) and cell production rate (change in cell density per day) from MPn treatments before day 25, after which cell concentrations began to decline. Figure 4: Pelagibacterales str. HTCC7211 produces methane when P i starved. ( a ) Total CH 4 concentration in sealed bottles from Pelagibacterales sp. str. HTCC7211 cultures grown with MPn or P i . Points are the mean CH 4 concentration±1.0 s.d. ( n =3) ( b ) Cell densities from bottles of Pelagibacterales sp. str. HTCC7211 cultures grown with no P i , MPn or P i . Cell counts for each treatment were obtained from single bottles used solely for cell counts. ( c ) The CH 4 production rate (change in CH 4 concentration per day) and cell production rate (change in cell density per day) from MPn treatments before day 25, after which cell concentrations began to decline. Full size image Table 1 CH 4 production by str. HTCC7211 from MPn (10 μ M) as a function of P i addition*. Full size table Table 2 Pelagibacterales sp . str. HTCC7211 cell yield as a function of added P. Full size table Table 3 Specific growth rates of str. HTCC7211 in AMS1 with varying levels of P i or MPn. Full size table Our data reveal a differential capacity for DOP utilization among the Pelagibacterales , with str. HTCC7211, but not str. HTCC1062, having a broad enzymatic capacity for DOP utilization ( Fig. 1 ). MPn was used by str. HTCC7211 in place of P i ( Fig. 1 ) and when doing so, CH 4 was stoichiometrically released ( Fig. 4 ). Consistent with these observations, genes encoding enzymes and transporters necessary to catabolize MPn (and other phosphonates) were upregulated under P i limitation ( Fig. 3 ). MPn hydrolysis was strongly repressed by P i ( Table 1 ), suggesting that in situ CH 4 production via MPn degradation by Pelagibacterales bacteria is likely to be confined to P i -deplete ocean regimes, such as the Sargasso Sea. Accordingly, published metagenomic analyses of multiple oceanic environments show that the Pelagibacterales -like C–P lyase genes are not universally distributed, but instead are more abundant in P i -deplete waters [13] , [14] , [15] . Although Pelagibacterales are likely to contribute meaningfully to the observed CH 4 supersaturation in surface waters because of their large population size, calculating their specific contribution is challenging owing to the uncertainties pertaining to strain heterogeneity with respect to C–P lyase gene content and how that may relate to the observed niche partitioning of Pelagibacterales ecotypes. In the Sargasso Sea, total Pelagibacterales cell abundances oscillate between 0.5 and 2.2 × 10 8 cells l −1 with maximum abundances at or above the pycnocline [40] . Spatiotemporal variation in the distribution of Pelagibacterales ecotypes has been discussed in multiple studies [31] , [40] , [41] . The degree to which the presence of C–P lyase genes correlates with the different Pelagibacterales ecotypes and whether the relative abundances of Pelagibacterales -like C–P lyase genes fluctuate seasonally is unknown. When analysing pyrosequences from the Sargasso Sea, Martinez et al. [13] showed that 82.5% of the identifiable phnI genes (used as a proxy for the presence of the C–P lyase) best hit to str . HTCC7211’s phnI gene, suggesting that Pelagibacterales members mediate a large portion of the C–P lyase activity in the Sargasso Sea. Using a metric called ‘multiplicity per cell,’ Coleman and Chisholm [14] analysed metagenomic data from the Sargasso Sea (collected in October of 2006) and calculated that ~\n52% of all Pelagibacterales cells contained phnJ , a marker gene used to infer the presence of the C–P lyase gene suite [16] . Multiplying the approximate abundance of C–P lyase containing Pelagibacterales cells found in the P-deplete Sargasso Sea (52%, based on phnJ , of 0.5–2.2 × 10 8 cells l −1 ) by the maximal net cell-specific CH 4 production rate measured here (0.42 amol CH 4 per cell per day; Fig. 4 ), we estimate maximal CH 4 production potential of ca. 0.01–0.05 nM per day via MPn hydrolysis. As MPn is part of a complex milieu of dissolved organophosphorus compounds that Pelagibacterales can use (for example, those illustrated in Fig. 1 ), the actual CH 4 production rates are probably much lower than the potential contribution calculated above. In situ CH 4 production rates are probably a function of (i) MPn supply relative to the total bioavailable DOP pool accessible to the Pelagibacterales ; (ii) the relative efficiency with which MPn is used when multiple substrates are simultaneously available; and (iii) the percent of the Pelagibacterales population that contain C–P lyase genes. We speculate that maximal CH 4 production by Pelagibacterales may occur shortly after the seasonal spring mixing event in the Sargasso Sea. This hypothesis is consistent with the observation that MPn producers (ammonia-oxidizing MGI archaea) are most active at 120 m, the base of the euphotic zone in the Sargasso Sea [42] , and that Pelagibacterales stocks increase sharply after spring mixing [40] . The laboratory results presented here help to contextualize metagenomic [13] , [14] , [15] and metaproteomic [38] findings that suggested that Pelagibacterales bacteria actively transport and use DOP, including phosphonates and P-esters, in the Sargasso Sea ( Fig. 1 ). The significance of these findings is extended to the global climate by showing that P i -starved Pelagibacterales produce CH 4 when MPn is provided as a sole P source ( Fig. 4 ). Interestingly, in addition to the abundant MGI archaea, some Pelagibacterales ecotypes may also harbour genes encoding the MPn synthase enzyme [18] , suggesting Pelagibacterales may also be an MPn source in the ocean. An understanding of environmental MPn dynamics (including supply and consumption rates) as it pertains to DOP utilization, remains a significant challenge to resolving CH 4 fluxes as they pertain to P stress in marine environments. Although methane production by P i -starved bacterioplankton is a probable source of CH 4 in P i -deplete waters rich in MPn, there may be other CH 4 -producing biological pathways that bear consideration. For example, in the nitrate-deplete, P i -replete waters of the central Arctic Ocean, an inverse correlation between CH 4 and a common resource for bacterial carbon and sulphur, dimethylsulphoniopropionate (DMSP), was found [27] . In subsequent incubation experiments, when DMSP was added to the Arctic surface waters, CH 4 was produced and α - and γ -proteobacteria increased in relative abundance [27] . From these results, Damm et al. [27] hypothesized a type of ‘methylotrophic methanogenesis’ in which the methylated degradation products of DMSP (methanethiol in particular) act as a precursor for CH 4 production. Although this is an intriguing possibility that may represent an alternate, and potentially significant, CH 4 source in aerobic surface waters, the enzymes, pathways and organisms involved have not yet been identified. Further study of mechanisms of aerobic CH 4 production in relationship to bacterial diversity and gene expression are needed to further unravel oceanic CH 4 sources. Organism source ‘ Candidatus Pelagibacter ubique’ str. HTCC1062 (ref. 43 ) and Pelagibacterales sp. str. HTCC7211 (ref. 32 ) were revived from 10% glycerol stocks and propagated in artificial seawater medium for SAR11 (AMS1) [39] , without added P i , but amended with pyruvate (100 μM), glycine (5 μM), methionine (5 μM), FeCl 3 (1 μM), and vitamins (B 1 : 6 μM; B 3 : 800 nM; B 5 : 425 nM; B 6 : 500 nM; B 7 : 4 nM; B 9 : 4 nM; B 12 : 700 pM; Myo-inositol: 6 μM; 4-aminobenzoate: 60 nM). P sources were added as indicated through the main text. Cultivation details All cultures, except those describing CH 4 production (described below), were grown in acid-washed and autoclaved polycarbonate flasks. Cultures were incubated at 20 °C with shaking at 60 r.p.m. under a 12-h light:12-h dark cycle. Light levels during the day were held at 140–180 μmol photons m −2 s −1 . Cells for cell counts were stained with SYBR green I and counted with a Guava Technologies flow cytometer at 48–72 h intervals as described elsewhere [44] . The treatments for the alternate phosphate source utilization experiments were: no P i addition (negative control), 1.0 μM P i (as NaH 2 PO 4 ; positive control), 1.0 μM phosphite (as NaPHO 3 ·5H 2 O), 1.0 μM glucose 6-phosphate, 1.0 μM ribose 5-phosphate, 1.0 μM MPn, 1.0 μM 2-aminoethylphosphonic acid or 1.0 μM phosphoserine. All alternate phosphorus compounds were ≥98% pure. Methane production from MPn Pelagibacterales sp . str. HTCC7211 cells, previously grown in media with MPn as the sole P source, were used to inoculate sterile, BSA-coated glass serum bottles containing growth media amended with 10 μM MPn as the sole P source. The negative control consisted of str. HTCC7211 cells, previously grown in media with P i as the sole P source, as inoculum for sterile, BSA-coated serum bottles containing growth media amended with 10 μM P i as the sole P source. Serum bottles (60 ml) were filled with 55 ml culture, leaving a 5-ml headspace, capped with Viton septa, crimped with aluminum seals and incubated horizontally in the conditions described in ‘Cultivation details.’ Cell counts for each treatment were obtained from single bottles used solely for cell counts. CH 4 in the headspace was measured by gas chromatography using a Shimadzu GC-8A gas chromatograph equipped with a column packed with Porapak N (80/100 mesh size) fitted with a flame ionization detector. In brief, 100 μl samples of headspace from each bottle were injected into the GC at a flow rate of 25 ml min −1 using ultrapure helium (He) as the carrier gas. Peaks were integrated using PeakSimple chromatography software ( http://www.srigc.com/ ). Quantification of CH 4 was accomplished by calibrating peak areas to the flame ionization detector response to a three-point calibration conducted at the beginning and end of the experiment using 100 μl injections of 100, 1,000 and 10,000 p.p.m. CH 4 standards. The 1,000 and 10,000 p.p.m. standards were prepared from a 1% mixed gas standard containing CH 4 , ethane and ethylene. Replicates of the 100 p.p.m. standard were analysed alongside samples on each sampling day. Over the course of the experiment, the peak area for the 100 p.p.m. standard varied by <5% (coefficient of variation). Headspace equilibration models at 20 °C using a Bunsen coefficient of 0.0345 for a 60 ml total volume (55 ml liquid, 5 ml headspace) suggest the fraction of the methane in the gas phase to be 74.5%. The fractionation of CH 4 between headspace and aqueous phase was verified by injecting commercial CH 4 standards (1.0 ml of either 100 p.p.m. or 10,000 p.p.m. CH 4 equivalent to 4.08 nmol CH 4 , 40.8 nmol CH 4 and 408 nmol CH 4 , respectively) into sealed serum bottles containing uninoculated growth medium. Of the added CH 4 , 72±6% in these standards was measured in the headspace at 20 °C. A value of 74% was used to adjust headspace CH 4 measurements to total CH 4 . Dissolved phosphorus measurements Samples for determination of total dissolved P levels were obtained at the end of CH 4 bioassays (see ‘Methane production from MPn ’) . Cells were removed from spent growth medium by filtration through a 0.02-μm Acrodisc filter. The dissolved inorganic P (DIP) concentration of the filtrate was determined colorimetrically as described by Murphy and Riley [45] using a Cary ultraviolet–visible spectrophotometer. The total dissolved P concentration of the filtrate was measured using a modification [19] of the Valderrama method [46] . Briefly, samples were oxidized at 120 °C for 60 min in Teflon digestion bombs, allowed to cool and run as DIP, as described above. The oxidizing agent used was a solution of potassium persulphate, sodium hydroxide and boric acid (as per ref. 46 ) added in a 1:10 oxidant to sample ratio. DOP concentrations were calculated as the difference between total dissolved P and DIP. Microarray growth and sampling conditions Biological replicates ( n =3) of str. HTCC1062 or str. HTCC7211 were grown in AMS1 (ref. 39 ) amended with pyruvate (1 mM), glycine (50 μM), methionine (50 μM), FeCl 3 (1 μM), P i (10 μM) and vitamins (as described above). In mid- to late-logarithmic growth ( ca. 0.7-1.0 × 10 8 cells ml −1 ), cells were harvested by centrifugation (17,664 g for 1.0 h at 20 °C). Cell pellets were evenly split and washed twice with growth media that was either amended with 100 μM P i (replete conditions) or not amended with P i (deplete conditions). After washing, pellets were re-suspended in P i -deplete or P i -replete growth media. Samples were collected from cell suspensions at t =0, 4, 20 and 38 h after resuspension for str. HTCC1062, and t =0, 20, 38, 68 and 96 h after resuspension for str. HTCC7211. Sampling consisted of centrifugation (48,298 g for 1.0 h at 4 °C) followed by resuspension of cell pellets in ‘RNAprotect Bacteria’ reagent (Qiagen, Valencia, CA). RNA was extracted using an RNeasy Mini kit (Qiagen) and amplified using the MessageAmp-II Bacteria RNA amplification kit (Ambion, Carlsbad, CA) using the manufacturer’s instructions. Amplified and labelled RNA was hybridized to custom ‘ Candidatus Pelagibacter ubique’ Affymetrix GeneChip arrays (Pubiquea520471f) (Affymetrix, Santa Clara, CA) that contained probes for Pelagibacterales strains HTCC1002, HTCC1062 and HTCC7211 as described previously [47] . Briefly, Affymetrix GeneChip arrays were hybridized and scanned using an Affymetrix GeneChip fluidics station, hybridization oven and scanner. Background and raw expression values were normalized between chips using the robust microarray algorithm using the Affymetrix Expression Console software. A Bayesian statistical analysis was conducted using Cyber-T [48] . The estimate of variance was calculated in Cyber-T by using window sizes of 101 and a confidence value of 10. A t -test was performed on log -transformed expression values by using the Bayesian variance estimate. The programme QVALUE, was used to obtain a q -value, which accounts for multiple t -tests performed [49] . A gene was defined as differentially expressed if both the q -value was ≤0.05 and the gene was differentially regulated by ≥2.0-fold. Accession codes: The raw microarray data files are deposited in the NCBI Gene Expression Omnibus (GEO) database with accession codes GSM1318808 to GSM1318861 . How to cite this article: Carini, P. et al. Methane production by phosphate-starved SAR11 chemoheterotrophic marine bacteria. Nat. Commun. 5:4346 doi: 10.1038/ncomms5346 (2014).